A family of transposable elements co-opted into developmental enhancers in the mouse neocortex The neocortex is a mammalian-specific structure that is responsible for higher functions such as cognition, emotion and perception. To gain insight into its evolution and the gene regulatory codes that pattern it, we studied the overlap of its active developmental enhancers with transposable element (TE) families and compared this overlap to uniformly shuffled enhancers. Here we show a striking enrichment of the MER130 repeat family among active enhancers in the mouse dorsal cerebral wall, which gives rise to the neocortex, at embryonic day 14.5. We show that MER130 instances preserve a common code of transcriptional regulatory logic, function as enhancers and are adjacent to critical neocortical genes. MER130, a nonautonomous interspersed TE, originates in the tetrapod or possibly Sarcopterygii ancestor, which far predates the appearance of the neocortex. Our results show that MER130 elements were recruited, likely through their common regulatory logic, as neocortical enhancers. Transcriptional enhancers control when, where and how much of each gene is produced in different cell types at different times [1] . Together, groups of enhancers orchestrate the expression of many genes to form complex pathways, but a fundamental question is what produced this coordinated regulatory logic. Instances of recognizable transposable element (TE) families make up more than half the human genome [2] , providing a large substrate of homologous sequences on which evolution can act. Britten and Davidson [3] proposed a mechanism by which the evolution of novel structures or functions could be greatly accelerated through the co-option of TEs into gene regulatory roles, activating novel groups of genes that were not co-expressed before in a new temporally and spatially specific manner. By scattering copies of the same DNA stretches across the genome near all manner of genes, TEs could greatly increase the probability that groups of enhancers would emerge to bring together a new group of genes, to be expressed together and accelerate the formation of complex new pathways and functions. Consistent with the idea of TEs seeding regulatory sequences, TEs have contributed significantly to conserved non-coding elements, via their co-option into gene regulatory roles [4] . In addition, TE families have been co-opted in different contexts such as stem cells [5] and the placenta [6] . p300 is a transcriptional co-activator recruited by active enhancers. It is an appealing epigenomic mark of active enhancers, with typical in vivo validation rates of 80% (ref. 7 ). In a recent paper [8] , we measured the p300 landscape of the E14.5 dorsal cerebral wall (DCW), which encompasses and gives rise to the neocortex, by harvesting tissue from mouse embryos, isolating chromatin and performing chromatin immunoprecipitation followed by high-throughput sequencing (ChIP-seq). In that study, we used multiple techniques to validate the quality of our p300 measurements, including confirming key enhancers known from the literature and enrichment analysis showing that from thousands of measured tissue-time-point combinations, our set is most correlated with genes expressed in Theiler stage 22 telencephalon (essentially E14.5 DCW). Using transgenics, we confirmed that eight of ten (80%) p300 measurements function as active neocortical enhancers, and established a primary cortical neuron transfection system where 5/8 positive transgenics showed transfection activity and 2/2 negative transgenics did not [8] . Here we show that the MER130 repeat family is strongly enriched among the E14.5 enhancers in the developing neocortex, an enrichment that is specific to mouse brain tissues. MER130 is a nonautonomous interspersed repeat family that previously has been shown to be conserved in mammals and chicken [9] . In pursuit of the Britten and Davidson [3] hypothesis, we show that the activity of MER130 family members is the result of a preserved core of regulatory logic that consists of multiple transcription factor binding sites. Individual MER130 instances function as enhancers, although we show that endogenous chromatin state is essential for interpreting these results. Furthermore, MER130 instances that function as enhancers lie next to important cortical genes, yet are conserved to species that far predate the emergence of the neocortex. MER130 is highly enriched among neocortex enhancers Intrigued by the Britten and Davidson [3] hypothesis and encouraged by the high specificity of the p300 mark, we asked whether any of ~1,000 known TE families are disproportionately marked by an in vivo p300-bound set of active enhancers (see Methods). One repeat family in one specific context stood out ( Fig. 1a ): MER130 in the E14.5 DCW with a 73-fold enrichment over expected (Bonferroni P value<0.006, n =1,000,000 simulations) [8] . 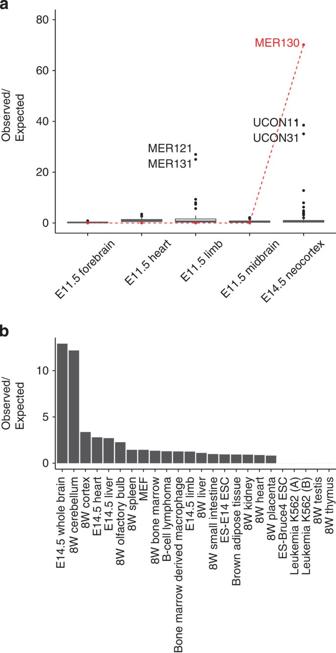Figure 1: MER130 is strongly enriched among neocortical enhancers. (a) Fold enrichments compared with uniform shuffles for over 1,000 interspersed repeat families among p300 ChIP-seq data sets from developing tissues. MER130 enrichments in red. (b) Fold enrichment of observed MER130 instance overlaps compared with expected overlaps from uniform shuffles of 24 ENCODE H3K27ac sets, including different primary tissues at different developmental time points and model cell lines. No enrichment comes close to the E14.5 neocortex enrichment ina. Figure 1: MER130 is strongly enriched among neocortical enhancers. ( a ) Fold enrichments compared with uniform shuffles for over 1,000 interspersed repeat families among p300 ChIP-seq data sets from developing tissues. MER130 enrichments in red. ( b ) Fold enrichment of observed MER130 instance overlaps compared with expected overlaps from uniform shuffles of 24 ENCODE H3K27ac sets, including different primary tissues at different developmental time points and model cell lines. No enrichment comes close to the E14.5 neocortex enrichment in a . Full size image Interestingly, MER130 was not enriched in any of the number of other p300-bound sequences from ChIP-seq experiments in other tissues, including the forebrain at an earlier time point ( Fig. 1a ). The histone modification H3K27ac, deposited by p300 at active enhancers [10] , is easier to assay and is thus a more comprehensively surveyed mark. We next searched for MER130 activity in multiple additional tissues by performing the same enrichment test for H3K27ac ChIP-seq sets from all 24 available tissues and cell lines from the mouse Encyclopedia of DNA Elements (ENCODE) [11] . We saw only weaker enrichments in other brain tissues: 12.9-fold enrichment for E14.5 whole brain, 12.2-fold for 8-week cerebellum, and <4-fold enrichment in non-brain tissues ( Fig. 1b ). Together, these data show a strong enrichment for MER130 in E14.5 DCW, with more modest enrichment in general brain tissue, compared with over 20 other tissue-time-point combinations. MER130 instances preserve a core regulatory logic We next comprehensively annotated the MER130 family using nhmmer, a probabilistic alignment tool [12] (107 instances; Supplementary Table 1 ; see Methods). Essentially all of the MER130 instances are distal (>2.5 kb from the transcription start site), and, as opposed to some other repeat families [13] , none overlap protein coding exons. We identified 23 well-conserved MER130 instances that were strongly enriched for the p300 ChIP-seq signal but not enriched for the input control signal (see Methods). Fourteen MER130 instances also overlap E14.5 whole-brain H3K27ac ChIP-seq peaks: eight strongly marked by p300 in our set and six marked with intermediate levels of p300. No instance marked by low levels of p300 in our set was marked by H3K27Ac in E14.5 whole brain. To achieve their specificity, enhancers contain distinct combinations of transcription factor binding sites [14] . When we constructed a multiple alignment from the 23 MER130 instances strongly enriched for p300 signal, it revealed a well-conserved ~100 bp core ( Fig. 2b ) containing 5 putative transcription factor binding sites resembling motifs from our library [15] , [16] : a Neurod/Neurog motif, an Nfi dimer [17] and two additional Nfi sites ( Fig. 2a ), representing families of factors important for brain development (see Discussion section). 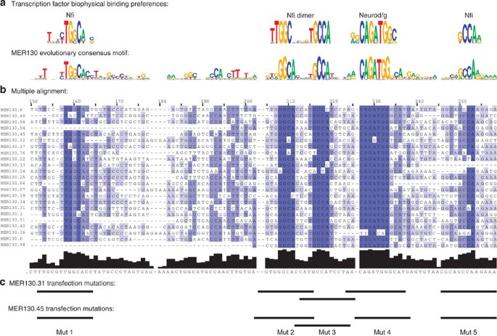Figure 2: MER130 contains a preserved core of transcriptional regulatory logic. (a) Biophysical transcription factor binding preferences (top) and matching consensus motif (bottom) derived from multiple alignment of MER130 instances marked by p300. (b) Multiple alignment of 23 MER130 instances strongly enriched for p300 signal. (c) Bases mutated in transfections (seeFig. 4). Figure 2: MER130 contains a preserved core of transcriptional regulatory logic. ( a ) Biophysical transcription factor binding preferences (top) and matching consensus motif (bottom) derived from multiple alignment of MER130 instances marked by p300. ( b ) Multiple alignment of 23 MER130 instances strongly enriched for p300 signal. ( c ) Bases mutated in transfections (see Fig. 4 ). Full size image p300-marked MER130 instances function as enhancers Next, we used our primary cortical neuron transfection system to test whether the MER130 instances marked by p300 functioned as enhancers and whether the binding sites preserved in the multiple alignment were necessary for their activity (see Methods). We cloned each of these 23 elements upstream of a minimal promoter and luciferase reporter, and transfected these constructs into dissociated neurons isolated from E14.5 mouse cortices (see Methods). Twenty-two of twenty-three (95.7%) of the MER130 candidates hypothesized to function as neocortex enhancers produced greater than twofold expression relative to the empty vector ( Fig. 3a , Supplementary Fig. 1 ). 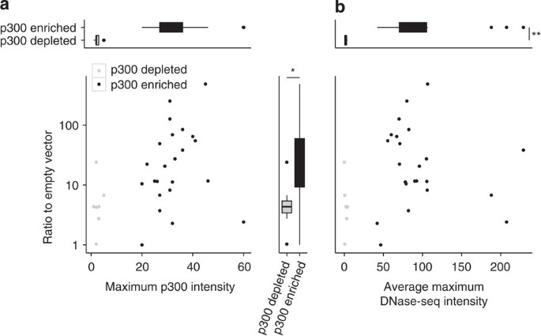Figure 3: MER130 members function as enhancers but may not occupy open chromatin. (a) Maximum neocortex p300 ChIP-seq intensity (x-axis) plotted against average fold activity relative to the empty vector when transfected into dissociated cortical neurons (y-axis) for each MER130 instance tested. (b) Average DNase-seq intensity across two mouse E14.5 whole-brain replicates (x-axis) plotted against samey-axis as (a) for the same set of MER130 instances. In both panels, MER130 elements enriched for the p300 signal in black (n=23) and depleted for the p300 signal in grey (n=7).t-test. *Pvalue<0.05; **Pvalue<0.01. Figure 3: MER130 members function as enhancers but may not occupy open chromatin. ( a ) Maximum neocortex p300 ChIP-seq intensity ( x -axis) plotted against average fold activity relative to the empty vector when transfected into dissociated cortical neurons ( y -axis) for each MER130 instance tested. ( b ) Average DNase-seq intensity across two mouse E14.5 whole-brain replicates ( x -axis) plotted against same y -axis as ( a ) for the same set of MER130 instances. In both panels, MER130 elements enriched for the p300 signal in black ( n= 23) and depleted for the p300 signal in grey ( n= 7). t -test. * P value<0.05; ** P value<0.01. Full size image Our result confirms that the MER130 instances marked by p300 function as enhancers. While virtually all MER130 instances preserve the 5 binding site core ( Supplementary Fig. 2 ), over half (56 instances, 52%) of MER130 instances are clearly devoid of a DCW p300 mark (the remainder show weak overlap, below our peak-calling threshold; see Methods). We cloned seven instances most depleted for p300 signal and tested them in the same transfection assay. Six of seven (85.7%) of these MER130 instances drove greater than twofold expression relative to the empty vector, though at a significantly weaker level than the set marked by p300 (p300 enriched, n =23, to p300 depleted, n= 7, t -test P value: 0.03; fold: 8.5) ( Fig. 3a , Supplementary Fig. 1 ). To better understand the in vivo state of these sequences, we examined the chromatin state from mouse E14.5 whole-brain DNase-seq data. Remarkably, the MER130 instances that were not marked by p300, yet functioned as enhancers in dissociated cortical neurons, were significantly (p300 enriched, n =23, to p300 depleted, n =7, t -test P value: 3.9e−09; fold: 51.7) depleted for DNase I cleavage when compared with the p300-marked MER130 instances that functioned in transfection assays ( Fig. 3b ). Of the 107 MER130 instances we annotate in the mouse genome, 103 (96%) are conserved to human. We explored the chromatin state of these conserved instances in day 85 human foetal brain tissue from the Roadmap Epigenomics Project [18] . Day 87 is the human time point matched to cortical neurogenesis in E14.5 mice [19] . Strikingly, MER130 instances not marked by p300 occupied closed chromatin not only in mouse, but also in human brain ( Supplementary Fig. 3 ). We then tested the necessity of the preserved core for driving specific expression levels in dissociated cortical neurons. Of the p300-enriched MER130 instances robustly expressed in our transfection assay and preserving the five binding sites, we chose two at random. We mutated each of the 5 preserved binding sites in these 2 MER130 neocortex enhancers ( Fig. 2c ) and tested the resulting 10 constructs in our primary cortical neuron transfection system. Mutating 7/10 (70%) predicted binding sites in the two enhancers resulted in a significant reduction (wild-type to mutant fold change of 1.8–7.7) of reporter activity ( Fig. 4 ). 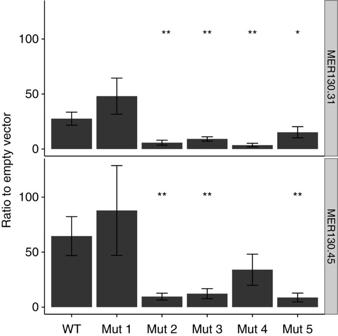Figure 4: MER130 core mutations modulate enhancer activity similarly across different instances. Two MER130 instances were mutated each at five putative binding sites (nomenclature as inFig. 2c). Average fold activity relative to the empty vector when mutated MER130 instances were transfected into dissociated cortical neurons. Error bars represent s.d.n=3 biological replicates × 3 technical replicates for each condition.t-test. *Pvalue<0.05; **Pvalue<0.01. All five pairs trend in the same direction, with 7/10 mutations significantly reducing expression. Figure 4: MER130 core mutations modulate enhancer activity similarly across different instances. Two MER130 instances were mutated each at five putative binding sites (nomenclature as in Fig. 2c ). Average fold activity relative to the empty vector when mutated MER130 instances were transfected into dissociated cortical neurons. Error bars represent s.d. n =3 biological replicates × 3 technical replicates for each condition. t -test. * P value<0.05; ** P value<0.01. All five pairs trend in the same direction, with 7/10 mutations significantly reducing expression. Full size image MER130 instances near critical neocortical development genes To identify functional coherence among the genes putatively regulated by the MER130 neocortex enhancers, we analysed them with GREAT [20] , a genomic region enrichment tool. We did not observe any statistically significant enrichments for either the full set of 107 MER130 elements or the set of 22 validated MER130 neocortex enhancers. Six of twenty-two validated MER130 cortical enhancers, however, do reside next to genes whose perturbations result in abnormal telencephalon morphology: Robo1 , Id4 , Dgkb , Ap3b1 , Prok2 and Zfp423 . We also observed a second MER130 instance marked by intermediate levels of p300 adjacent to two of these six genes: Robo1 and Zfp423 . From the remaining MER130 instances not enriched for p300 at E14.5, we observe MER130 instances next to eight additional genes annotated with abnormal telencephalon morphology: Cadm1 , Enah , Epha4 , Foxg1 , Mycn , Npas3 , Park2 and Pax3 (ref. 21 ). MER130 originated in or before the tetrapod ancestor The MER130 family is likely an interspersed repeat due to its consensus length (~470 bp), composition and distribution across the genome [13] . We queried all known repeat families and databases of RNAs but found no homologous sequences that may help shed light on the identity of MER130 (see Methods). We also searched 75 vertebrate genome drafts and found no species with recent MER130 activity ( Supplementary Table 2 and Methods). While MER130 was previously thought to originate in the amniote ancestor [9] , we discovered that in fact it is conserved in Xenopus tropicalis , suggesting this element originated no later than the tetrapod ancestor ( Fig. 5a ). We also identified a single possible ancestral match in the Coelacanth genome ( Fig. 5c ). This hit occurs in the NRF1 orthologue, a gene that mediates neurite outgrowth [22] . Interestingly, despite the weak sequence conservation, this coelacanth element drives greater than twofold activity when tested in dissociated cortical neurons ( Fig. 5b ). No MER130 matches were found in seven species of bony fish or lamprey. 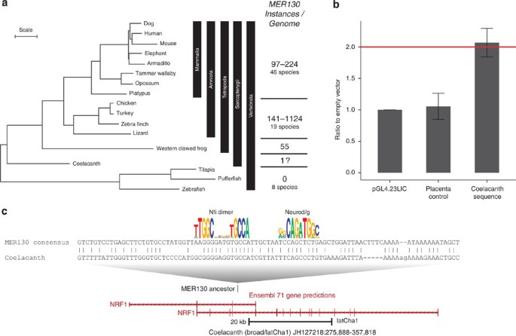Figure 5: MER130 originated in the tetrapod or Sarcopterygii ancestor. (a) Phylogenetic tree (adapted from ref.43) with representative species and the range of MER130 instances in species from each clade. Scale, 0.1 substitutions per site. (b) Average fold activity relative to the empty vector when the coelacanth sequence (c) was transfected into dissociated cortical neurons. Error bars represent s.d. (c) Alignment between Dfam MER130 model and Coelacanth genomic locus. Aligning bases preserve Nfi dimer and Neurod/g motifs (Fig. 2). The putative MER130 instance in coelacanth is located in an intron ofNRF1, a gene that mediates neurite outgrowth. Figure 5: MER130 originated in the tetrapod or Sarcopterygii ancestor. ( a ) Phylogenetic tree (adapted from ref. 43 ) with representative species and the range of MER130 instances in species from each clade. Scale, 0.1 substitutions per site. ( b ) Average fold activity relative to the empty vector when the coelacanth sequence ( c ) was transfected into dissociated cortical neurons. Error bars represent s.d. ( c ) Alignment between Dfam MER130 model and Coelacanth genomic locus. Aligning bases preserve Nfi dimer and Neurod/g motifs ( Fig. 2 ). The putative MER130 instance in coelacanth is located in an intron of NRF1 , a gene that mediates neurite outgrowth. Full size image Forebrain expression of genes near MER130 instances Finally, we used the fact that MER130 is not present in fish to ask whether the appearance of a MER130 instance next to a tetrapod gene makes it more likely to be expressed in the forebrain than its orthologue in fish. Using the GREAT default gene-region association rule, our 22 active MER130 instances can be associated with 37 immediately adjacent genes. Seventeen of these genes, adjacent to 13 MER130 instances, are annotated with ‘TS21–TS23 forebrain expression’ in GXD [21] . Of the same 37 genes, we map 28 to orthologous genes in zebrafish using the Ensembl orthologue mappings. Nineteen of these are annotated for gene expression in any context in ZFIN [23] , and of them, only 3 genes are annotated for forebrain expression. While anecdotal, these results suggest that new gene expression domains in the developing neocortex are associated with the emergence of the MER130 family. The 73-fold enrichment of co-opted MER130 elements among E14.5 DCW enhancers is striking. Similar magnitude enrichments have previously only been reported in the context of embryonic stem cells [5] , [24] , with maximal folds in the twenties for non-ES cell types or lines [6] , [24] . When we examined the MER130 elements, we observed a clear core whose pattern of preservation recapitulates the known biophysical binding preferences of two important transcription factor families. The common activation code of Neurod/g and Nfi binding sites are the likely reason for their recruitment as a transcriptional network of neocortical enhancers. Together, these features represent a striking example in support of the Britten and Davidson [3] hypothesis. Neurog and Nfi family members are promising candidates for transcriptional regulators of MER130, given that Neurog2 -mutant mice, as well as mice null for Nfia , Nfib and Nfix , all exhibit abnormal telencephalon morphology, the same phenotype exhibited by mice null for multiple putative MER130 target genes [25] , [26] , [27] , [28] . The developing neocortex has been microdissected at E14.5 to isolate the three layers present at this time point, and gene expression in all three layers has been measured using RNA-seq [29] . Among Neurog family members, Neurog2 is the most highly expressed in all three layers at E14.5, and among Nfi family members, Nfib is the most highly expressed in all three layers. Both genes are in the first percentile of all expressed genes at this time point. The presence of four different Nfi binding sites in the MER130 consensus further supports its importance [30] . While our experiments suggest that most MER130 instances are capable of driving activity in the cortex, likely by virtue of their shared code, the MER130 instances marked by p300 at E14.5 drive higher relative activity when transfected in dissociated cortical neurons. In contrast with the constructs we tested in vitro , endogenous enhancer activity also depends on the chromatin state [31] . The lack of DNase I cleavage in both mouse and human brains suggests that the MER130 instances not bound by p300 in our measurements are not only weaker drivers in cortical neurons due to their sequence, but also likely not accessible in their endogenous context. MER130 is more ancient than previously thought. Our search of multiple vertebrate genomes places its origin at least as early as the common ancestor of tetrapods, and possibly as early as our common ancestor with coelacanth. The MER130 family exhibits an LF-SINE-like evolutionary behaviour, where exapted copies shed revealing 5′ and 3′ marks, leaving behind what is very likely only the body of the co-opted transposon [13] . We did not identify any instances co-opted into coding exons, suggesting MER130 may not have ended in a poly-A tail [13] . The sequencing of additional tetrapod genomes, especially genomically isolated ones, may yet reveal a species with a recently jumping copy, allowing for the classification of this repeat family [32] . All repeats—p300 sets correlation We downloaded the RepeatMasker track from the pre-annotated mm9 genome (RepeatMasker open-3.2.8 Repeat Library) [33] and removed low-complexity, satellite and simple repeat classes, while retaining DNA, LINE, SINE, LTR and RNA classes for a total of 1,118 repeat and RNA families. We next downloaded p300 ChIP-seq results for E11.5 forebrain [34] , midbrain, heart and limb [35] , and removed proximal peaks (<2.5 kb away from any transcription start site in UCSC knownGene track). We shuffled each p300 set across the genome 10,000 times (excluding the UCSC mm9 gap track). For each p300 set shuffle, we counted the number of p300 set instances overlapped by each repeat family. We also computed the number of actual p300 set instances overlapped by each repeat family. Fold enrichment was computed as observed divided by mean for each repeat family—p300 set combination. To better estimate the P value for the enrichment of the MER130 family and determine statistical significance, we performed an additional 1,000,000 shuffles of our neocortex p300 set against this repeat family alone. Tissue specificity We downloaded all 24 available H3K27ac tissue and cell-line data from ENCODE and removed all peaks overlapping an exon (UCSC mm9.knownGene) and proximal peaks (<2.5 kb away from any transcription start site). Observed and expected overlaps were computed as above. MER130 instances identification and intersection with p300 We used nhmmer (from hmmer3.1-snap20121011 using --cut-ga threshold) [12] to identify 107 instances of the MER130 repeat family in the mouse genome (NCBI37/mm9), using Dfam’s MER130 DF0000726.2 profile HMM model [2] . Each MER130 instance was semi-automatically classified as high, medium or low confidence based on computing maximum p300 signal intensity over each peak, followed by manual inspection. Read pileups were constructed using MACS1.4, and the maximum peak height was extracted using UCSC bigWigAverageOverBed. Maximum p300 read pileup from the p300 ChIP-seq was used as the primary selection attribute, and instances classified as high confidence had a punctuated peak over the MER130 family member, as well as low input control signal. This resulted in 23 well-conserved MER130 instances with maximum p300 read pileup height ≥20 (high), 28 instances marked by intermediate levels of p300 (7 ⩽ p300 ⩽ 24; medium) and 56 instances marked by background levels of p300 (0 ⩽ p300 ⩽ 6; low). Multiple alignment Sequences aligning to the DFAM DF0000726.2 profile HMM model (corresponding to the 23 MER130 instances strongly enriched for p300 signal) were extracted from the mouse genome (NCBI37/mm9). A multiple alignment of these sequences was then constructed using MUSCLE (v3.8.31; ref. 36 ). Ethics All animal work was carried out in compliance with the Stanford University Institutional Animal Care and Use Committee under approved protocols #18487 and #21758. Timed pregnant female mice were adults >6 weeks of age and maintained on a Swiss Webster background (Charles River). Embryos at the time of harvest were 14.5 days post coitum. Cloning and transfections Cloning and transfections were performed as in ref. 15 . Briefly, inserts were amplified from mouse genomic DNA (Clonetech Laboratories Inc.) using Phusion High Fidelity DNA Polymerase (NEB Inc.). For transfections using the coelacanth match to the MER130 consensus, a 196 bp insert containing the MER130 core match was amplified from coelacanth ( Latimeria menadoensis) genomic DNA. A Ligation Independent Cloning (LIC) site was ligated to the firefly luciferase vector, PGL4.23 (Promega Corp.), at the 5′ KpnI and 3′ HindIII sites, and all inserts were cloned into the PGL4.23 LIC vector using an LIC method [37] . All positive clones were identified by colony PCR and sequenced. E14.5 embryos were harvested from Swiss Webster mice (Charles River). The dorsal telencephalon was removed and stored briefly on ice in a Hank’s balanced salt solution dissection solution. Cells were dissociated using 0.25% trypsin and 10 μg μl −1 DNase. Nucleofections were performed using the experimental luciferase construct and a pRL-CMV Renilla control (Promega) and a P3 Primary Cell 96-well Nucleofector Kit (Lonza). Nucleofected cells were plated onto poly-D-lysine coated 96-well plates (NUNC) containing PNBM (Lonza). Luciferase assays were performed 48 h after nucleofection using the Dual-Luciferase Reporter 1000 Assay System (Promega) according to the manufacturer’s protocol and read using a Promega Glomax luminometer. An enhancer sequence that drove activity in placental cells, but not in cortical neurons in luciferase reporter assays [38] , was used as a negative control. Primers are listed in Supplementary Table 3 . Site-directed mutagenesis Site-directed mutagenesis was performed as in ref. 39 . Briefly, the PGL4.23 LIC vector containing the normal insert served as the template for short cycle PCR using specially designed primers and Phusion High Fidelity DNA Polymerase. DpnI was used to digest the template. All clones were identified by colony PCR and sequenced. Primers are listed in Supplementary Table 3 . Chromatin state Day 85 human foetal brain tissue DNase-seq intensities were downloaded from the Roadmap Epigenomics Project [18] . Mouse sequences were lifted to human using the UCSC liftOver tool (-minMatch=0.2), and the maximum peak height was measured using UCSC bigWigAverageOverBed. Genomic region enrichment analysis Enrichment analysis was performed using GREAT ( http://great.stanford.edu/ ) version 2.0.2 (ref. 20 ) with default parameters. MER130 origins and activity Sequences were queried using nhmmer [12] (from hmmer3.1-snap20121011 using --cut-ga threshold) with the Dfam [2] MER130 DF0000726.2 profile HMM model. We first searched the RepBase catalogue of repeats [9] to identify homologous repeat families, as well as the eukaryotic tRNA database [40] and Rfam [41] to probe for RNAs from which a SINE element may have been derived [13] . We then downloaded vertebrate genome sequences from UCSC ( http://hgdownload.cse.ucsc.edu/downloads.html ) and vertebrate scaffolds from Genbank Release 196 ( ftp://ftp.ncbi.nlm.nih.gov/genbank/genomes/Eukaryotes/vertebrates_other/ ). A total of 75 available vertebrate genome drafts were searched. We observed repeat densities of 0.0–0.5 copies per Mb ( Fig. 5a , Supplementary Table 2 ). The green sea turtle, with the highest repeat density of a modest 0.5 copies per Mb, had 1,124 MER130 copies present in its genome ( Fig. 5a , Supplementary Table 2 ). However, these instances were quite diverged from each other, suggesting that MER130 has long been inactive in this lineage as well [13] , [42] . How to cite this article: Notwell, J. H. et al. A family of transposable elements co-opted into developmental enhancers in the mouse neocortex. Nat. Commun. 6:6644 doi: 10.1038/ncomms7644 (2015).